New evidence suggests pyroclastic flows are responsible for the remarkable preservation of the Jehol biota The lower Cretaceous Yixian and Jiufotang formations contain numerous exceptionally well-preserved invertebrate, vertebrate and plant fossils that comprise the Jehol Biota. Freshwater and terrestrial fossils of the biota usually occur together within some horizons and have been interpreted as deposits of mass mortality events. The nature of the events and the mechanisms behind the exceptional preservation of the fossils, however, are poorly understood. Here, after examining and analysing sediments and residual fossils from several key horizons, we postulate that the causal events were mainly phreatomagmatic eruptions. Pyroclastic density currents were probably responsible for the major causalities and for transporting the bulk of the terrestrial vertebrates from different habitats, such as lizards, birds, non-avian dinosaurs and mammals, into lacustrine environments for burial. Terrestrial vertebrate carcasses transported by and sealed within the pyroclastic flows were clearly preserved as exceptional fossils through this process. The lower Cretaceous Yixian and Jiufotang formations occupy a volcanic terrane in western Liaoning, extending northwards to south-eastern Inner Mongolia and southwards to northern Hebei, and have yielded numerous completely preserved specimens of plants, insects, aquatic invertebrates, fishes, frogs, salamanders, turtles, lizards, choristoderes, pterosaurs, non-avian dinosaurs, birds and mammals that comprise the Jehol Biota [1] , [2] . Most of the specimens show various aspects of exceptional preservation, ranging from clear impressions of the body outlines to traces of soft tissues (for example, teleost air sac, eye spots, muscles, skin) and external body coverings (for example, scales, feathers, hairs) [2] , [3] . The biota, spanning the Barremian to early Aptian ( ca . 130–120 Ma) of the early Cretaceous [4] , [5] , is one of the most important Mesozoic Konservat-Lagerstätten in the world [3] , [6] . Fossils of both freshwater and terrestrial organisms typically occur together within single horizons, which have been interpreted as the result of mass mortality events [2] , [6] , [7] , [8] . The cause of these events has been generally attributed to frequent volcanic eruptions in the terrane because most fossiliferous strata are interbedded with 0.5–5 cm thick tuff layers [7] , [8] , [9] . In contrast, systematic excavations and examination of the sedimentary rocks reveal that most vertebrate and invertebrate fossils are preserved within extremely thin laminae (less than 1 mm) of lacustrine tuffaceous mudstones and tuffs. The fossiliferous laminae have no direct contact with the interbedded tuff layers that were interpreted as deposits from volcanic eruptions [6] , [10] , [11] . This finding led to the hypothesis that seasonal limnic overturn was responsible for the fossil concentrations [6] , [11] . However, several key issues regarding the process of fossilization remain unresolved. These include the cause of death of the terrestrial organisms that lived in diverse habitats in the region, the mechanism of transportation of their carcasses into a mixed graveyard and the preponderance of fully articulated fossils. The skeletons of terrestrial vertebrates and their enclosing sediments from the strata that formed during the mass mortality events contain key clues for answering these questions. Here we collect matrix rock samples of fourteen bird and non-avian dinosaur specimens from five of the most fossiliferous localities of the Jehol Biota ( Fig. 1 ), six of them comprising fragmental fossils. By examining and analysing the fossils and sediments, we untangle the exceptional preservation mechanism behind the biota. 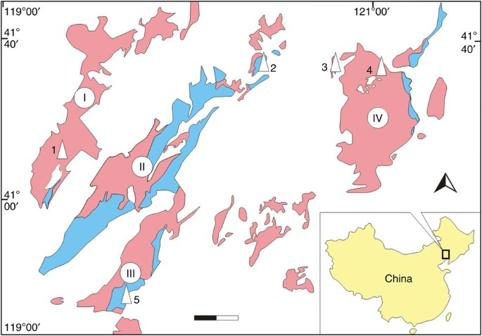Figure 1: Localities of the studied samples in western Liaoning. Distributions of the Yixian and Jiufotang formations are indicated in red and blue, respectively. I, Lingyuan-Sanshijiazi basin; II, Kazuo-Chaoyang basin; III, Jianchang basin; IV, Fuxin-Yixian-Jinzhou basin. Fossil localities: 1, Dangwangzhangzi of Lingyuan; 2, Shangheshou of Chaoyuang; 3, Sihetun of Beipiao; 4, Hejiaxin of Yixian; 5, Jiangchang. The arrow points to north and the scale bar is 20 km. The map is modified from ref.13. Figure 1: Localities of the studied samples in western Liaoning. Distributions of the Yixian and Jiufotang formations are indicated in red and blue, respectively. I, Lingyuan-Sanshijiazi basin; II, Kazuo-Chaoyang basin; III, Jianchang basin; IV, Fuxin-Yixian-Jinzhou basin. Fossil localities: 1, Dangwangzhangzi of Lingyuan; 2, Shangheshou of Chaoyuang; 3, Sihetun of Beipiao; 4, Hejiaxin of Yixian; 5, Jiangchang. The arrow points to north and the scale bar is 20 km. The map is modified from ref. 13 . Full size image The fossil-bearing lacustrine deposits Many lakes were developed in close association with active volcanoes in the terrane during Early Cretaceous time when the Jehol biota was formed. The lakes and volcanism developed during approximately four temporally and spatially overlapping phases ( Fig. 2 ). 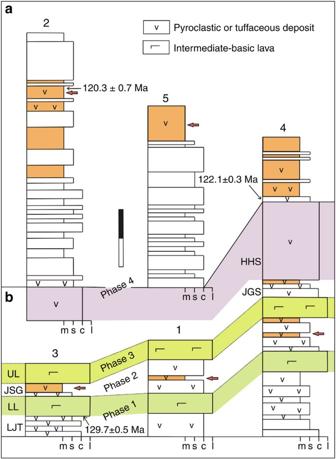Figure 2: Stratigraphic logs. Jiufotang (a) and Yixian (b) formations in the five studied localities. These sections show the distributions of thin-laminated lacustrine deposits (orange), sampling sites (red arrows), radiometrically dated horizons and interpreted phases of volcanism of the region. The scale bar represents 200 m. The sections are modified from ref.13. LJT, Lujiatun unit; LL, Lower Lava unit; JSG, Jianshangou unit; UL, Upper Lava unit; JGS, Jingangshan bed; HHS, Huanghuashan bed. Figure 2: Stratigraphic logs. Jiufotang ( a ) and Yixian ( b ) formations in the five studied localities. These sections show the distributions of thin-laminated lacustrine deposits (orange), sampling sites (red arrows), radiometrically dated horizons and interpreted phases of volcanism of the region. The scale bar represents 200 m. The sections are modified from ref. 13 . LJT, Lujiatun unit; LL, Lower Lava unit; JSG, Jianshangou unit; UL, Upper Lava unit; JGS, Jingangshan bed; HHS, Huanghuashan bed. Full size image The earliest three phases are best preserved in the volcanic succession of the lower part of the Yixian formation in the Sihetun area [12] . Initially, shield volcanoes developed with only minor volcaniclastic deposits (the Lujiatun unit and its equivalent strata), but extensive basaltic and andesitic lavas form the Lower Lava unit. The shield volcano phase terminated with explosive eruptions, resulting in many depressions such as craters and calderas. These depressions subsequently developed into volcanic lakes and partially filled with lacustrine deposits that form the Jianshangou unit and its equivalent strata. Frequent explosive eruptions apparently occurred adjacent to these lakes during this phase as evidenced by numerous tuff layers in the lacustrine deposits. The next phase was characterized by extensive lava flows and domes that form the Upper Lava unit. The last phase was dominated by more explosive eruptions, which formed the thick subaerial pyroclastic deposits (the Huanghuashan bed and its equivalent stratum of the upper part of Yixian Formation in Fig. 2 ) and numerous tuffaceous layers in the neighbouring lacustrine deposits (the Jingangshan bed of the upper part of Yixian Formation and the Jiufotang Formation in Fig. 2 ) [2] , [13] . Most of the Jehol fossils were collected from lacustrine deposits, with the exception being some vertebrates, which were locally recovered from volcaniclastic alluvial deposits of the Lujiatun unit and its correlative horizons [12] . The lacustrine deposits are characterized by thin-laminated tuffaceous mudstones and tuffs intercalated with thin-bedded tuffs or tuffaceous sandstones. Although terrestrial vertebrate fossils have been encountered throughout the lacustrine succession, most of them were concentrated and collected from extremely thin laminae of tuffaceous mudstones and tuffs ( Supplementary Fig. 1 ) [7] , [8] . The laminae have been interpreted as the result of suspension loads and turbidity currents in thermally stratified lacustrine environments [10] , [14] . Detailed excavations of the lacustrine deposits in the Sihetun area have revealed that the laminae are either non-fossiliferous or contain a lacustrine fauna with highly abundant specimens but low diversity. Three species dominate: the conchostracan Eosestheria ovata , the shrimp Liaoningogriphus quadripartitus and nymphs of the mayfly Hexagenites trisetalis . Each of these taxa dominates an assemblage, in that one species usually accounts for 85 to 98% of all individuals [6] , [11] . The plan-view orientation of these taxa is invariably random, and size-frequency histograms are bimodal or polymodal. The fauna has been interpreted as being autochthonous, reflecting the ‘background’ limnic fauna [12] and, thus, the deposits resulted from local mass mortalities [6] . In contrast, the terrestrial vertebrates that have been found throughout the depositional area of the lake floors represent outsiders introduced by catastrophic events [12] . Each fossiliferous layer usually contains several kinds of terrestrial vertebrates with an uneven areal density of specimens. In one area where over a thousand individuals of the same taxon, Confuciusornis , accumulated, the average density is about one specimen per 5–6 m 2 , with the highest density reaching one specimen per 1–2 m 2 locally [7] , [8] . Cause of the mass mortality events The layers containing terrestrial vertebrates are 5–10 mm thick and consist of planar laminae from 0.03 to 1 mm thick that are laterally discontinuous and internally structureless. They undulate subtly, tend to thicken in topographic lows and thin with finer-grain size over the crests of undulations. Locally, some laminae disappear into underlying layers and have the appearance of low-angle cross-lamination. Subspherical vesicles (gas bubbles) up to 50 μm in diameter commonly occur in the laminae. All the enclosing sediments are poorly sorted, and platy grains are aligned roughly parallel to bedding surfaces ( Fig. 3 ; Supplementary Figs 2–7 ). Carbonized plant fragments are common in the sediments, ranging from millimetres to tens of centimeters in size ( Supplementary Fig. 8 ). Viewed with the stereomicroscope, the plant debris display well preserved anatomic features covered by thin layers of fragmented black streaks on surfaces ( Supplementary Fig. 9 ). These features indicate carbonization of the plant fragments, most probably caused by charring [15] , [16] . 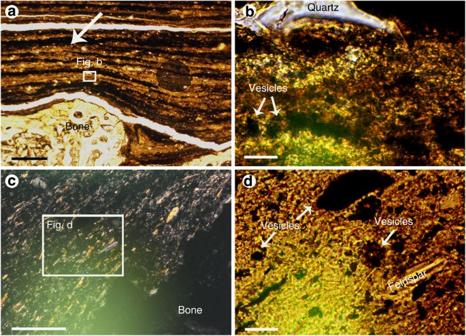Figure 3: Sedimentary features of the enclosing tuffs. Photomicrographs show subtly waved, planar-lamination in sediments overlying the skeletons of aPsittacosaurus(a,b) and aConfuciusornis(c,d). (a) The overview shows some laminae truncating others with a subtle erosional surface (arrow), poor sorting and parallel alignment of platy fragments to bedding surfaces. (b) A magnified view of the square area in (a) indicates the dominance of partly altered, extremely fine-grained vitric chips in the sediments. (c) The overview illustrates parallel alignment of platy grains to bedding surfaces and distinction of vitric shards. (d) A close-up view of the square area in (c) shows the dominance of partly altered, extremely fine-grained vitric chips in the sediment. Images (a,b,d) are with plane-polarized light and image (c) is taken with cross-polarized light. Scale bars:a, 500 μm;b, 20 μm;c, 100 μm;d, 20 μm. SeeSupplementary Figs 2–6for additional sedimentary structures. Figure 3: Sedimentary features of the enclosing tuffs. Photomicrographs show subtly waved, planar-lamination in sediments overlying the skeletons of a Psittacosaurus ( a , b ) and a Confuciusornis ( c , d ). ( a ) The overview shows some laminae truncating others with a subtle erosional surface (arrow), poor sorting and parallel alignment of platy fragments to bedding surfaces. ( b ) A magnified view of the square area in ( a ) indicates the dominance of partly altered, extremely fine-grained vitric chips in the sediments. ( c ) The overview illustrates parallel alignment of platy grains to bedding surfaces and distinction of vitric shards. ( d ) A close-up view of the square area in ( c ) shows the dominance of partly altered, extremely fine-grained vitric chips in the sediment. Images ( a , b , d ) are with plane-polarized light and image ( c ) is taken with cross-polarized light. Scale bars: a , 500 μm; b , 20 μm; c , 100 μm; d , 20 μm. See Supplementary Figs 2–6 for additional sedimentary structures. Full size image With polarized-light microscopy and scanning electron microscopy (SEM), we found that all the examined sediments that contain fossils are composed dominantly of extremely fine-grained vitric shards and pumice fragments, minor crystals of quartz, feldspar and mica, and lithic fragments. The vitric shards and pumice commonly show a degree of montmorillonitization and silicification. Particle sizes range from less than 1 μm to 150 μm in diameter. Larger particles (20–150 μm) are mainly composed of pumice, non-vesicular to poorly vesicular to blocky vitric shards with adhering dust, and grains of feldspar and quartz. Smaller particles (less than 20 μm) consist of moss-like masses of angular and irregular vitric chips ( Fig. 3 ; Supplementary Figs 2–7 ). X-ray diffraction (XRD) analyses (microdiffraction) of the particles taken directly from the surfaces of the six studied skeletons show that the sediments consist dominantly of quartz, K-feldspar (microcline and sanidine), muscovite and montmorillonite ( Supplementary Fig. 10 ). The fact that the sediments are primarily pyroclastic in origin without significant epiclastic components suggests that the skeletons were buried within primary tuffs. The tuffs bear characteristics of phreatomagmatic eruption products, such as extremely fine grain sizes (mostly <60 μm), blocky and moss-like grain shapes of vitric shards and pumice fragments, and the common occurrence of vesicles in the laminae [17] , [18] , [19] . Various sedimentary features of the tuffs, including very poor sorting, erosion into underlying laminae, wavy layering, lateral discontinuity and trapping of grains within lows of the laminae layering and parallel alignment of platy grains to bedding surfaces, all suggest that the sediments enveloping the skeletons resulted from base surges, which are characteristic of pyroclastic density currents (PDCs) from phreatomagmatic eruption [19] . If so, the accompanying charcoalified plant fragments were probably derived from charring caused by hot, dry phreatomagmatic eruptions that produced base surges that engulfed terrestrial plants, a common feature of PDC deposits [15] , [16] . The lower parts of the surges may have transformed into subaqueous density flows when they pushed their way across the lake water and emplaced deposits indistinguishable from their subaerial counterpart. This would be similar to what is thought to have happened when the PDCs of the 1883 Krakatau eruption entered the sea [20] . The direct embedding of all the examined specimens within PDC deposits indicates that the Jehol animals, belonging to different vertebrate groups, were probably killed when pulses of nearby phreatomagmatic eruptions occurred close to the lakes where the carcasses became entombed. The eruptions must have been numerous and caused multiple mass mortalities of both terrestrial and aquatic animals in the region, as do contemporary explosive eruptions [21] . Death and burial of the animals The possibility that the terrestrial animal remains were carried into lacustrine environments by surface water can be ruled out. There are two ways to transport entire carcasses via surface water into a thermally stratified lake provided they survived intact until they reached the lake’s interior: either by floating all of the way into the lake or by being carried by turbidity currents triggered by input of floods. In the former case, the carcasses would have been covered by deposits of the water’s suspended load, so that the resulting laminae would have been laterally continuous as commonly observed in lacustrine deposits of suspended sediments [10] , [14] . This mode of deposition is not consistent with the features of the tuff laminae that we observed. In addition, preservation of highly articulated vertebrate skeletons is not supported by the hypothesis of long-distance floating of the carcasses because the skeletons would not come to rest on the lake floor until significant disarticulation had occurred, as taphonomic experiments on birds have showed [22] . In the scenario of the turbidity current transport, the carcasses would be embedded in graded, epiclastic or reworked pyroclastic sediments rather than the internally structureless laminae of primary tuffs that enclose the studied specimens. Distal turbidity currents producing laminae up to 1 mm thick must be of low energy and could not transport skeletons of various vertebrates. There are three alternative explanations of how animals died and were carried to the lake floor during phreatomagmatic eruptions: air blasts generated by explosive eruptions, avian species falling from the sky or incorporation into PDCs. Explosive air blasts would break up most of the carcasses and distribute them with a strongly decreasing gradient in quantity from the vent [23] , which does not match the preservation conditions and extensive distributional patterns of the skeletons found in the studied lacustrine deposits. Accidental falling of birds can be easily conceived: they encountered eruptions when flying over lakes, and were suffocated by gases and fell into lakes, as observed at the city of St Pierre during the 1902 Mount Pelée eruptions in West Indies [24] . Such sky dropping may explain the fate of some birds but not that of other vertebrates associated with the birds. Of these three explanations, our data best support the mechanism involving capture and transport of terrestrial animals in PDCs. Numerous Jehol specimens of mammals, feathered non-avian dinosaurs and birds show entombment poses of limb flexure, that is, limbs flexed and spine extended ( Supplementary Fig. 11 ) [25] , [26] , [27] , [28] , [29] , [30] , [31] , [32] . The limb flexures of the skeletons are typical postures of PDC victims, which result from postmortem shortening of tendons and muscles [33] , [34] . Statistical documentation of head–tail axes of Confuciusornis carcasses revealed a distinct orientation (E–W) [7] , [12] , which is consistent with the preferred orientation of victims of PDCs, such as seen in the 1902 Mount Pelée eruptions [33] . In addition, most Jehol terrestrial vertebrate skeletons lie either on their sides or ventrodorsally with their largest surface more or less parallel to bedding. As observed in many other specimens, cross-sections across bones from two of the studied skeletons show that the underlying laminae are asymmetrically deformed, whereas the overlying layers are evenly capped ( Supplementary Fig. 12 ). The asymmetrical deformation of the underlying laminae resembles the bedding sag structure that is formed by impact of ballistic ejecta upon beds capable of being plastically deformed in base surge deposits of phreatomagmatic eruptions [19] . The asymmetric deformation suggests that the carcasses were transported in a specific direction and dropped onto the lake floor. This interpretation accords with the capacity of PDCs to carry their victims and drop their remains far away from where they were engulfed [24] . Furthermore, evidence for charring and thermal modification exists in all six studied skeletons. The skeletons are commonly enveloped in a thin dark layer, which forms a two-dimensional body outline. Similar to the coating sediments, XRD analysis of particles taken from the dark layer covering a Confuciusornis skeleton shows that the material is composed of quartz and orthoclase/sanidine ( Supplementary Fig. 13 ). SEM and SEM-based energy dispersive X-ray (EDS) analyses on bone surfaces and thin sections of the six studied skeletons reveal that the dark layer contains abundant carbonaceous materials. The materials are constituted of poorly to well preserved, open cell structure, the walls of which are shiny, polygonally fragmented or cracked, vacuolated and locally homogenized. These features indicate that the materials are probably carbonized muscular, dermal and epidermal tissues. Extremely fine-grained pyroclasts or pyroclastic aggregates are directly in contact with or locally fill tubular structures within the layers, which were possibly blood vessels or other lumina in the original soft tissues ( Fig. 4 ; Supplementary Figs 14–17 ). We did not detect any precipitated authigenic mineral phase aggregated in or surround the cell structures, which is required for duplication of soft tissues during fossilization [35] , [36] . Carbonized soft tissues have not been observed from the accompanying, aquatic Jehol fossils in this study ( Supplementary Fig. 18 ) or in previous reports [14] , [37] . Thus, the carbonized soft tissues of the terrestrial vertebrates cannot be explained as the degraded remains of original tissues. Instead, they bear characteristic features of charcoals, such as an open cell structure, thin cell walls and vacuolated, partly-homogenized polygonal cracks [15] . The direct contact of the soft tissues with pyroclastics indicates that the charring was caused by hot-emplaced volcanic ash, a characteristic common for victims of PDCs [33] , [38] . 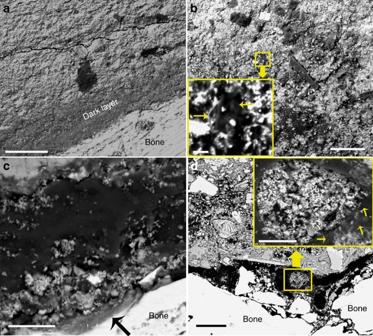Figure 4: Charcoalified soft tissues. (a,b) Backscattered environmental SEM images on thePsittacosaurusskeleton. (a) This polished cross-section through a rib shows the dark layer and the black fragments overlying on it. (b) A close-up view of the femur surface shows preservation of possible cell structures (arrows in the inset image). (c,d) Backscattered SEM images of a carbon-coated, thin section through a leg of theConfuciusornisskeleton. (c) Blackened, homogenized soft tissues with filling of vitric chips. Note also the presence of blackened upper edge of the bone (arrow). (d) Poorly preserved but discernible, partly homogenized open cell structures (arrows in the inset image) in tubular structures, possibly blood vessel and lumina of the soft tissues. Scale bars:a, 100 μm;b, 100 μm and 10 μm (inset);c, 5 μm;d, 20 μm and 5 μm (inset). Figure 4: Charcoalified soft tissues. ( a , b ) Backscattered environmental SEM images on the Psittacosaurus skeleton. ( a ) This polished cross-section through a rib shows the dark layer and the black fragments overlying on it. ( b ) A close-up view of the femur surface shows preservation of possible cell structures (arrows in the inset image). ( c , d ) Backscattered SEM images of a carbon-coated, thin section through a leg of the Confuciusornis skeleton. ( c ) Blackened, homogenized soft tissues with filling of vitric chips. Note also the presence of blackened upper edge of the bone (arrow). ( d ) Poorly preserved but discernible, partly homogenized open cell structures (arrows in the inset image) in tubular structures, possibly blood vessel and lumina of the soft tissues. Scale bars: a , 100 μm; b , 100 μm and 10 μm (inset); c , 5 μm; d , 20 μm and 5 μm (inset). Full size image Partially exposed bone surfaces of the studied skeletons are also carbonized ( Fig. 4 ; Supplementary Fig. 14 ). XRD analysis shows that bones of all the six studied skeletons are preserved as a cryptocrystalline intergrowth of hydroxylapatite-fluorapatite solid solution and quartz and that the hollow parts of the Confuciusornis bones are filled with precipitated quartz ( Supplementary Figs 13 and 19 ). Thin sections of two studied skeletons show that the haversian lamellae are well preserved in the spongy and inner part of compact bones. The lamellae become poorly defined but discernible towards the outer compact layer and vanish at bone edges. Cracks spreading outwards from haversian canals are common with fine crisscrossed cracks visible at bone edges ( Supplementary Fig. 20 ). Asymmetrical wavy abrasive pits, which commonly result from losses of bones alone cracks or osteons, occur at both the upper and lower bone edges. Accordingly, bone debris is commonly found in the adjacent embedding sediments ( Supplementary Fig. 15 ). Carbonized bone surfaces, cracks spreading outwards from haversian canals, fine crisscrossed cracks at bone edges and microstructure absent towards bone surfaces are comparable to features from victims at Pompeii and nearby archaeological sites caught in PDCs from the 79 AD eruption of Mt. Vesuvius [34] . Similarly, these characteristics are consistent with experimental results from heating modern bones [34] , [39] . The asymmetrically wavy abrasive pits on bone surfaces and loss of bone debris into embedding sediments may result from heat erosion during transport in PDCs as the susceptibility of bones to fragmentation is known to significantly increase after their being heated [39] . These features suggest that the Jehol terrestrial animals were engulfed by PDCs and then charred, transported and deposited onto the lake floor, as is observed with modern day volcanic eruptions [24] , [33] . Mechanism for exceptional preservation The mechanism by which PDCs captured, transported and buried animals explains the exceptional preservation of diverse terrestrial vertebrates at Jehol. The fine-grained volcanic ash that encloses the remains probably formed moulds around complete skeletons, resembling the intact, buried corpses at Pompeii [33] , [40] . Rapid deposition of extremely fine-grained ash into thermally stratified lakes could have protected the remains from being scavenged and bioturbated and resulted in preservation of most articulated carcasses [41] , [42] . Fresh, hot, dry, acid volcanic ash promoted burning, charring or mummifying of soft tissues [33] , which, as a result, became more resistant to decay and better preserved [43] . The burnt, charred or mummified organic tissues probably served as templates for the extremely fine-grained ashes that coated them, forming the two-dimensional body outlines as in the case of the Burgess Shale [41] . The other less or unaffected soft-tissues, however, may have undergone full degradation due to absence of rapid precipitation of authigenic minerals. Previously, the preservation of the Jehol vertebrates was generally attributed to frequent volcanic eruptions in the terrane based on the evidence that most fossiliferous strata are found interbedded with tuff layers [7] , [8] , [9] , but an in-depth study of the mechanism has not been conducted until now. The mechanisms behind the formation of the Jehol Biota are clearly complex. However, based on our detailed examination of the sedimentary, petrological and morphological evidence from 14 specimens from five fossil localities, we propose that PDCs were the cause. The most probable mechanism involves phreatomagmatic eruptions that produced hot, dry, ash, which concentrated in engulfing PDCs and lead to the mass mortalities as well as their transportation and ultimate preservation as the Jehol terrestrial vertebrate fossils. Although only some terrestrial vertebrate fossils were examined in this study, similar conclusions may be drawn regarding other terrestrial fossils contained in the studied horizons because these horizons appear to record the same events. PDCs are lethal to the organisms they entrain [21] , which is not age dependent, so as happens now happened then. Moreover, PDCs as an agent in the fossil record are potentially applicable to other examples of preserved biota in or closely associated with tuffaceous deposits or tuffs that resulted from frequent volcanic eruptions [44] , [45] , [46] , [47] , [48] . Samples The studied specimens were borrowed from the Sihetun Fossil Museum and the Institute of Vertebrate Paleontology and Paleoanthropology, Chinese Academy of Sciences (IVPP). Samples of fourteen terrestrial vertebrate specimens were removed from the rock matrix. Samples subject to destructive analysis were chosen so as to accurately record the preservation conditions while minimizing damage. All the specimens were sampled from layers rich with terrestrial vertebrates and, thus, should represent mass mortality events from five of the most productive fossil localities in western Liaoning. Among these specimens, five are from the Yixian Formation in the Sihetun area of Beipiao (Locality 3 in Figs 1 and 2 ), including three birds Confuciusornis (Shtn, PI-V-29[4] and V980620) and two dinosaurs Psittacosaurus (PI-V-26 [B] and PI-V-28) from the most productive Confuciusornis -bearing and dinosaur-bearing layers, respectively; two unnamed enantiornithine birds (V13872, V16064) and one bird Liaoxiornis (V12414)) are from the Yixian Formation in the Dawangzhangzi area of Lingyuan (Locality 1 in Figs 1 and 2 ); two unnamed enantiornithine birds (V12556, V17629) are from the Yixian Formation in the Hejiaxin area of Yixian (Locality 4 in Figs 1 and 2 ); two birds Confuciusornis (V12644 and V12647) are from the Jiufotang Formation in the Shangheshou area of Chaoyang (Locality 2 in Figs 1 and 2 ); one bird Yanornis (V16709) and an unnamed enantiornithine bird (V16071) are from the Jiufotang Formation in Jianchang (Locality 5 in Figs 1 and 2 ). Six samples (Shtn, PI-V-26 [B], V16064, V12556, V17629 and V12647) contain partly exposed skeleton fragments ( Supplementary Fig. 1 ). Sample preparation Encased skeletons were identified by CT scanning using the 2010 GE phoenix v|tome|x s240 system ( Supplementary Fig. 1 ). Polished cross-sections and thin sections were prepared for observation using a polarized-light microscope and scanning electron microscope equipped with back-scattered electron (BSE) detector and energy dispersive x-ray spectra detector (EDX). Pyroclasts were disaggregated by soaking small pieces of sample in weak acid (5% HCl) for SEM analysis. SEM, XRD and CT analyses were carried out in the American Museum of Natural History. Scanning electron microscopy SEM analysis utilized both a Zeiss EVO 60, which is an environmental SEM capable of operating in variable pressure mode, and a Hitachi S-4700 with field-emission electron source. Samples were coated with either carbon, for BSE and EDS study, or gold, solely for imaging. X-ray microdiffraction Small fragments (<1 mm across) of bone and contacting sediment were examined by X-ray microdiffraction (XRD) analysis using a Rigaku DMAX/RAPID microdiffraction system employing monochromatized Cu Kα X-rays. Phase identification of XRD data was made using JADE (MDI) software. How to cite this article: Jiang, B. et al . New evidence suggests pyroclastic flows are responsible for the remarkable preservation of the Jehol biota. Nat. Commun. 5:3151 doi: 10.1038/ncomms4151 (2014).